A sequence variant in humanKALRNimpairs protein function and coincides with reduced cortical thickness Dendritic spine pathology is a key feature of several neuropsychiatric disorders. The Rac1 guanine nucleotide exchange factor kalirin-7 is critical for spine morphogenesis on cortical pyramidal neurons. Here we identify a rare coding variant in the KALRN gene region that encodes the catalytic domain, in a schizophrenia patient and his sibling with major depressive disorder. The D1338N substitution significantly diminished the protein’s ability to catalyse the activation of Rac1. Contrary to wild-type kalirin-7, kalirin-7-D1338N failed to increase spine size and density. Both subjects carrying the polymorphism displayed reduced cortical volume in the superior temporal sulcus (STS), a region implicated in schizophrenia. Consistent with this, mice with reduced kalirin expression showed reduced neuropil volume in the rodent homologue of the STS. These data suggest that single amino acid changes in proteins involved in dendritic spine function can have significant effects on the structure and function of the cerebral cortex. In the mammalian forebrain, most excitatory synapses are located on dendritic spines, small protrusions of dendrites [1] . Spine morphology modulates synaptic properties and the ability to undergo plasticity [2] , [3] . Spine plasticity driven by changes in synaptic activity contributes to the remodelling of neural circuits during postnatal development, including experience-dependent plasticity which occurs throughout life. Spine enlargement parallels various forms of potentiation, including long-term potentiation, whereas long-term depression seems associated with spine shrinkage [4] . Accordingly, spines can undergo morphological changes in live animals following changes in sensory input and during social interactions, stress, environmental enrichment, learning and other behavioural conditions [5] . Abnormal synaptic connectivity is a well-established characteristic of several psychiatric disorders, including schizophrenia, but the exact molecular mechanisms underlying synaptic pathogenesis are not known [6] , [7] . Mounting evidence indicating that known schizophrenia susceptibility genes regulate spines strongly reinforces the hypothesis that perturbations in the molecular pathways underlying spine plasticity are deeply involved in the development and progression of schizophrenia [7] . Because dendrites and spines make up a significant fraction of the cortical neuropil, it has been hypothesized that changes in dendrite and spine number and morphology may lead to alterations in cortical thickness measures, a finding reported in several mental disorders, including schizophrenia [8] . Changes in the actin cytoskeleton are heavily implicated in the morphological alteration of spines and are controlled by proteins of the small GTPase family [9] . These proteins serve as molecular switches that fluctuate between GTP-bound active and GDP-bound inactive states, and are controlled by guanine nucleotide exchange factors (GEFs) and GTPase activating proteins [10] . One of these small GTPase regulators, the Rac-GEF commonly known as kalirin-7 but sometimes referred to as Duo, has been identified as both having a critical role in spine morphogenesis and associated with increased psychiatric risk [7] , [11] . Kalirin-7, encoded by the human KALRN gene and the rodent Kalrn gene, is the most highly expressed kalirin protein isoform in the adult rodent brain, with its highest expression levels in the cerebral cortex and hippocampus [12] , [13] . It is primarily localized to spines, and its expression levels rise during a period corresponding to that of synaptogenesis [12] , [14] . Kalirin-7 catalyses the activation of Rac1, thereby allowing it to bind to p21-activated kinase (PAK), which in turn facilitates actin remodelling [15] , [16] . Overexpression of kalirin-7 results in increased spine number [15] , and neurons in which kalirin-7 has been knocked down display reductions in spine density [17] . Kalirin-7 is also required for NMDA receptor-dependent structural plasticity and concomitant increases in synaptic AMPA receptor expression [17] , [18] and interacts with the products of schizophrenia susceptibility genes DISC1 (ref. 19 ), NRG1 and ERBB4 (ref. 20 ) to regulate spine and dendrite plasticity. Kalrn knockout mice display a periadolescent reduction in cortical dendritic spine number and reduced dendritic complexity, as well as deficits in working memory that emerge in adolescence [18] , [21] . KALRN has been associated with schizophrenia risk through resequencing and association analysis [22] and postmortem analyses of patients’ cortical KALRN mRNA and protein levels [23] , [24] . Recent large scale studies revealed that rare sequence variants, such as copy number variations and exonic mutations in glutamatergic synaptic plasticity genes are enriched in subjects with schizophrenia [25] , [26] . However, functional analyses of such sequence variants, especially exonic mutations, present in human subjects in synaptic plasticity genes have not been extensively performed. In addition, the relationship between such molecular and cellular variations and macroscopic brain morphometric phenotypes has not been examined. As an initial step in this direction, we sought to identify coding and potentially functionally important variants in KALRN in human subjects, assess the functional impact of such variations, and explore neuromorphometric parameters in carrier subjects. We thus sequenced specifically in the region that codes for the kalirin protein’s Rac1-GEF catalytic domain. We identified one such variant, which significantly impaired protein function and neuronal morphology. Interestingly, the subjects carrying this variant displayed reduced cortical thickness in the caudal portion of the superior temporal sulcus. Consistent with this, mice lacking the Kalrn gene show reduced cortical thickness, suggesting a potential link between molecular and cellular alterations and macroscopic neuromorphological phenotypes. Identification of KALRN sequence variants We screened for missense sequence variants in exons 23–28 of human KALRN ( Fig. 1a ), which encode the Dbl-homology (DH) portion of its gene products’ Rac1-GEF enzymatic domain, in a cohort of well-characterized schizophrenia subjects. Sequencing and automated indel/SNP analysis of these exons led to the identification of a rare coding variant, NC_000003.12:g.124462620G>A (NP_001019831.2:p.D1338N), located in the Rac1-GEF domain of KALRN in a single subject with schizophrenia (KAL-SCZ, Fig. 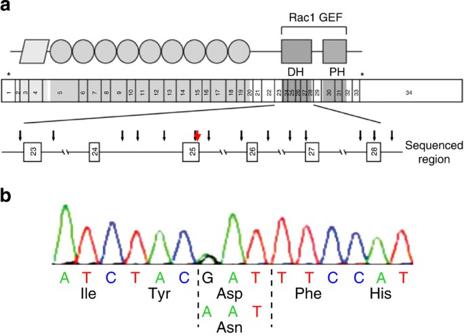Figure 1: Identification of theKALRNvariant coding for kalirin-7 p.D1338N. (a) Schematic of the kalirin-7 protein (top), mRNA (middle) and the genomic regions that were sequenced. The catalytic Rac1-GEF domain, composed of Dbl-homology (DH) and pleckstrin-homology (PH) domains, is indicated. Fourteen distinct silent and intronic variants identified among 127 patients are denoted by black arrows, and the SNP leading to the p.D1338N variant is denoted by a red arrow. (b) Chromatogram illustrating that KAL-SCZ is heterozygous for the minor allele (NC_000003.12:g.124462620G>A) responsible for the kalirin-7 coding variant. The chromatogram from KAL-SIB showed a similar result. 1b ; Supplementary Table 1 ). 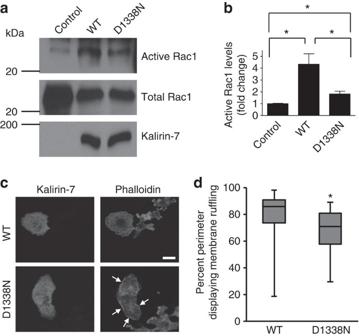Figure 2: Biochemical consequences of the D1338N variant. (a,b) Activation of Rac1 is attenuated in hEK-293 cells expressing kalirin-7-D1338N as compared with those expressing wild-type (WT) kalirin-7. Rac1-GTP was isolated by incubation of cell lysates with a GST-PAK binding domain fusion protein, and levels were normalized to total Rac1 and kalirin-7 expression. Three independent experiments were performed, each of which involved transfection of two wells of cells per condition. (c,d) COS-7 cells expressing myc-kalirin-7-D1338N (lower panels) exhibit a lesser degree of membrane ruffling, as visualized by staining with Alexa488-conjugated phalloidin, than do those expressing wild-type kalirin-7 (upper panels). The cell in the upper left panel displays ruffles on nearly 100% of its perimeter, whereas the cell in the lower left panel only displays ruffles in distinct locations (arrows). Analysis of 30–35 cells was performed for each condition. *P<0.05. Data are mean±s.e.m. Scale bar, 10 μm. This initial screen was followed by a second screen for the variant in siblings and non-diseased controls ( Supplementary Table 2 ). The only carrier for the variant identified in this screen was a sibling of KAL-SCZ (KAL-SIB), who although not schizophrenic, had been diagnosed with major depressive disorder and alcohol and cocaine dependence. This known minor allele (rs139954729) is predicted by PolyPhen [27] to be probably damaging, with a score of 0.981 (sensitivity: 0.75; specificity: 0.96). It was not found in European ancestry subjects in a large exome-sequencing data set, NHLBI GO Exome Sequencing Project (ESP) ( n =4,300; http://evs.gs.washington.edu/EVS/ ). It is also found in African American subjects ( n =4,404 chromosomes), but with a very low population frequency (0.044%). We could not establish the statistical evidence for the association with schizophrenia due to the limited sample size and incidence of the variant. Nevertheless, we sought to determine whether it would lead to cellular phenotypes, given that the variant was identified in a schizophrenia patient and his sibling with other neuropsychiatric disorders, as well as its low population frequency and the predicted deleterious property. Figure 1: Identification of the KALRN variant coding for kalirin-7 p.D1338N. ( a ) Schematic of the kalirin-7 protein (top), mRNA (middle) and the genomic regions that were sequenced. The catalytic Rac1-GEF domain, composed of Dbl-homology (DH) and pleckstrin-homology (PH) domains, is indicated. Fourteen distinct silent and intronic variants identified among 127 patients are denoted by black arrows, and the SNP leading to the p.D1338N variant is denoted by a red arrow. ( b ) Chromatogram illustrating that KAL-SCZ is heterozygous for the minor allele (NC_000003.12:g.124462620G>A) responsible for the kalirin-7 coding variant. The chromatogram from KAL-SIB showed a similar result. Full size image Biochemical characterization of the D1338N variant The p.D1338 residue is located in the Rac1-GEF domain of KALRN, and is highly conserved across species in related protein family members, so we hypothesized that a substitution that changes the charge from an acidic to a slightly basic residue in this domain is likely to affect protein function. To determine whether this would be the case, we transfected hEK-293 cells with a cDNA homologous to either the human major allele (referred to hereafter as ‘wild-type kalirin-7’) or D1338N kalirin-7 constructs and performed a Rac1 activation affinity assay ( Fig. 2a ; Supplementary Fig. 1 ). As expected, overexpression of wild-type kalirin-7 induced approximately a fourfold increase in Rac1-GTP levels compared with untransfected cells ( Fig. 2b ). While overexpression of the D1338N variant led to an increase in Rac1 activation as compared with the untransfected condition, the degree of activation was significantly less than that induced by wild-type kalirin-7. These results indicate that the D1338N kalirin-7 variant is impaired with respect to the protein’s ability to catalyse the exchange of GDP for GTP bound to Rac1. Figure 2: Biochemical consequences of the D1338N variant. ( a , b ) Activation of Rac1 is attenuated in hEK-293 cells expressing kalirin-7-D1338N as compared with those expressing wild-type (WT) kalirin-7. Rac1-GTP was isolated by incubation of cell lysates with a GST-PAK binding domain fusion protein, and levels were normalized to total Rac1 and kalirin-7 expression. Three independent experiments were performed, each of which involved transfection of two wells of cells per condition. ( c , d ) COS-7 cells expressing myc-kalirin-7-D1338N (lower panels) exhibit a lesser degree of membrane ruffling, as visualized by staining with Alexa488-conjugated phalloidin, than do those expressing wild-type kalirin-7 (upper panels). The cell in the upper left panel displays ruffles on nearly 100% of its perimeter, whereas the cell in the lower left panel only displays ruffles in distinct locations (arrows). Analysis of 30–35 cells was performed for each condition. * P <0.05. Data are mean±s.e.m. Scale bar, 10 μm. Full size image As many of the downstream effectors of Rac1 are known to cause remodelling of the actin cytoskeleton, we reasoned that a kalirin-7 variant that has impaired GEF activity would also be less able to stimulate actin polymerization. We have previously shown that membrane ruffling, a morphological indicator of actin polymerization, can be induced by expression of either full length kalirin-7 protein or the kalirin-7 GEF domain alone [14] . Therefore, we examined the effect of the D1338N variant on membrane ruffling in COS-7 cells ( Fig. 2c ). The majority of cells expressing wild-type kalirin-7 exhibited membrane ruffling along greater than 80% of their perimeters, representing a significantly greater degree of actin polymerization than that induced by kalirin-7-D1338N ( Fig. 2d ). Thus, the kalirin-7-D1338N variant’s diminished capacity for Rac1 activation has functional consequences in the context of cytoskeletal reorganization. Neuronal morphology in kalirin-7-D1338N expressing neurons The processes of dendritic spine maturation, excitatory synapse potentiation, and de novo spine formation are all dependent on remodelling of the actin cytoskeleton [3] , [28] . The requirement of kalirin-7 in regulating these processes in forebrain pyramidal neurons has been well established [11] , [13] . As such, we sought to determine whether the D1338N substitution would impair the ability of kalirin-7 to promote spine growth and development ( Fig. 3a ). In mature cortical pyramidal neurons (21–28 DIV), overexpression of kalirin-7-D1338N failed to enhance spine density and area, whereas wild-type kalirin-7 overexpression increased both spine parameters ( Fig. 3b ). These data indicate that the D1338N variant not only impacts kalirin-7 protein function, but also has severe effects on spine structural plasticity. 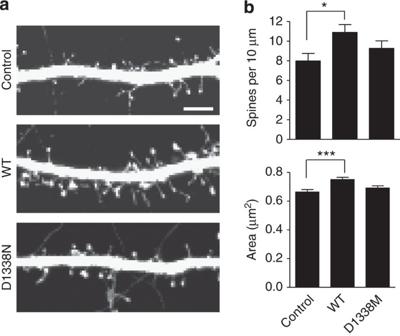Figure 3: Dendritic spine density and area following kalirin-7 transfection. (a) Rat cortical pyramidal neurons were transfected with an eGFP expression vector alone (top panel), or with wild-type kalirin-7 (middle panel) or kalirin-7-D1338N (bottom panel). (b) Quantification of spine density (upper panel) and spine area (lower panel) reveals an increase in both parameters in the neurons overexpressing wild-type kalirin-7. No change was seen following overexpression of kalirin-7-D1338N. *P<0.05; ***P<0.001. Data are mean±s.e.m. Scale bar, 5 μm. Figure 3: Dendritic spine density and area following kalirin-7 transfection. ( a ) Rat cortical pyramidal neurons were transfected with an eGFP expression vector alone (top panel), or with wild-type kalirin-7 (middle panel) or kalirin-7-D1338N (bottom panel). ( b ) Quantification of spine density (upper panel) and spine area (lower panel) reveals an increase in both parameters in the neurons overexpressing wild-type kalirin-7. No change was seen following overexpression of kalirin-7-D1338N. * P <0.05; *** P <0.001. Data are mean±s.e.m. Scale bar, 5 μm. Full size image MR imaging of D1338N carriers Spine morphology is thought to contribute to brain neuropil volume, and postmortem analyses and structural MR imaging studies of the brains of patients have provided evidence for reduced spine density and cortical thickness in the prefrontal and auditory association cortices in schizophrenia. To explore whether the subjects carrying the kalirin-7-D1338N variant displayed unique neuromorphometric features, we compared MRI measures of cortical thickness between the carrier subjects and noncarriers. This preliminary comparison suggested that both the subject with schizophrenia (KAL-SCZ) and the sibling with depression (KAL-SIB) had reduced cortical thickness in the posterior banks of the left superior temporal sulcus (STS) as compared with the means of comparison groups of schizophrenia subjects (SCZ), their unaffected siblings (SCZ-SIB), and control subjects (CON) ( Fig. 4a,b ). 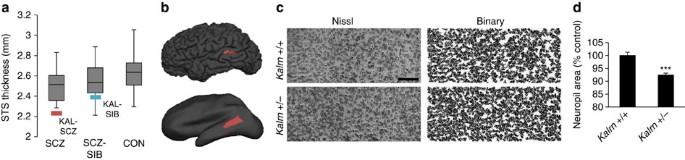Figure 4: Impact of kalirin-7 hypofunction on cortical thickness. (a,b) Both KAL-SCZ (red bar) and KAL-SIB (blue bar) had reduced cortical thickness in the left superior temporal sulcus (STS; location on pial and inflated surfaces illustrated in the upper and lower panels, respectively, ofb) as compared with the means of their respective experimental groups. The STS thickness measurement for KAL-SCZ was 1.72 s.d. lower than the SCZ group mean. (c,d) Quantification of neuropil area in the temporal association cortex of 12-week-old wild-type mice (c, upper panels) and litter-matched heterozygousKalrnnull mice (c, lower panels) revealed a reduction in neuropil in mice carrying only one functionalKalrnallele. Neuropil was calculated by performing Nissl staining (c, left panels), binarizing and filtering images of the tissue (c, right panels), and calculating the area of the images not occupied by neuronal somata. Eight to twelve images were acquired from each of the three or four animals per genotype. ***P<0.001. Data are mean±s.e.m. Scale bar, 100 μm. Figure 4: Impact of kalirin-7 hypofunction on cortical thickness. ( a , b ) Both KAL-SCZ (red bar) and KAL-SIB (blue bar) had reduced cortical thickness in the left superior temporal sulcus (STS; location on pial and inflated surfaces illustrated in the upper and lower panels, respectively, of b ) as compared with the means of their respective experimental groups. The STS thickness measurement for KAL-SCZ was 1.72 s.d. lower than the SCZ group mean. ( c , d ) Quantification of neuropil area in the temporal association cortex of 12-week-old wild-type mice ( c , upper panels) and litter-matched heterozygous Kalrn null mice ( c , lower panels) revealed a reduction in neuropil in mice carrying only one functional Kalrn allele. Neuropil was calculated by performing Nissl staining ( c , left panels), binarizing and filtering images of the tissue ( c , right panels), and calculating the area of the images not occupied by neuronal somata. Eight to twelve images were acquired from each of the three or four animals per genotype. *** P <0.001. Data are mean±s.e.m. Scale bar, 100 μm. Full size image Thinner cortex in Kalrn -deficient mice Because a causal relationship cannot be established in this case, we sought to determine whether reduced kalirin signalling in animal models could result in cortical morphological phenotypes consistent with the neuroimaging human phenotypes. We have previously reported that total knockout of the Kalrn gene in mice leads to reduced cortical thickness, as measured in the frontal cortex [18] , [21] . We therefore analysed cortical neuropil area in the secondary auditory and temporal association cortices of Kalrn heterozygote mice, which better mimic the reduced kalirin signalling of the kalirin-7-D1338N variant ( Fig. 4c ). We labelled cell bodies by perfoming Nissl staining on coronal sections from 12-week-old mice, and defined neuropil as the area of the tissue that was devoid of stain. Kalrn heterozygotes exhibited a significant reduction in neuropil area as compared with wild-types ( Fig. 4d , 92.4±0.8% of wild-type area). These data indicate the necessity of intact functional kalirin expression for normal cortical morphology. Recent genomic studies have revealed extensive interindividual variability and diversity in the human genome, including common and rare variants, missense and nonsense mutations and copy number variants [29] , [30] . Genome-wide association and copy number variation studies of schizophrenia and other psychiatric disorders have identified many new disease susceptibility genes involving both common single-nucleotide polymorphisms (SNPs) and rare disease variants, most of which contribute small effects [31] . In addition, variations in a number of genes have been associated with mental disorders such as schizophrenia [32] , [33] . It has been suggested that variations that increase risk for mental disorders cluster in gene networks that controls the synapse development and plasticity [34] . However, few studies have examined sequence variation in human genes encoding synaptic proteins, their molecular and cellular functional consequences, and their potential impact on human brain neuroimaging and phenotypes. In the current study, we have established the presence of a rare KALRN sequence variant in a patient–sibling pair, which results in a single amino acid change in the kalirin-7 protein’s catalytic GEF domain. Although we did not establish this variant as a risk for schizophrenia, it is predicted to be deleterious and present at a very low frequency in the human population. In addition, while the sibling carrying the variant did not present with schizophrenia, she had been diagnosed with major depressive disorder, the treatment of which has been linked to increased dendritic spine formation [35] . Pleiotropy is commonly seen in psychiatric disorders and other complex traits (reviewed in Duan et al. [31] ). A schizophrenia susceptibility locus may be associated with not only other psychiatric disorders [36] , [37] , but also some other nonpsychiatric disorders, such as multiple sclerosis [38] and cardiovascular-disease [39] . Among psychiatric disorders, such shared genetic susceptibility may be due to the shared subphenotypes. Symptoms of mood disorder are common among individuals with schizophrenia [40] , and they are also observed in their relatives at rates higher than those observed in the general population. In addition, in young adults, depression may be a prodromal sign of psychosis [41] . Moreover, variations in clusters of genes, including KALRN, implicated in schizophrenia and psychotic bipolar disorder aetiology may impact resting state functional activity in affected individuals and first-degree relatives. This attests to the impact of common and rare genetic variation on measurable functional outcomes potentially related to disease phenotypes [42] . One hypothesis for the minor allelic variant in KALRN would be that this variant alters cortical thickness, a subphenotype that manifests as schizophrenia or major depressive disorder depending on other genetic modifiers or different individual genetic backgrounds. At the cellular level the slightly altered protein affects phenotypes, particularly with regard to dendritic spines, in a manner similar to that of kalirin-7 proteins that lack a functional GEF domain [15] , as well as those which are incapable of being phosphorylated by upstream signalling proteins [17] . Therefore, it stands to reason that altered function in proteins in the kalirin-7 signalling pathway could also cause dendritic spine dysfunction, and, at the anatomical level, cortical thinning. It has previously been shown that kalirin-7 interacts with DISC1 (ref. 19) [19] , and that it is a necessary component of pathways downstream of both NRG1/ERBB4 and 5-HT2A serotonin receptors [43] , [44] . DISC1 variants associated with schizophrenia correlate with reduced cortical thickness in several regions independent of psychiatric diagnosis [45] , [46] . Knockdown of DISC1 in cultured cortical neurons also results in diminished dendritic spine number [19] , and frontal cortex pyramidal neurons in mice carrying DISC1 missense variants or truncations display reduced spine number and dendrite length than those in wild-types [47] , [48] . Similarly, patients carrying a schizophrenia-associated minor NRG1 allele have reduced superior temporal gyrus volumes as compared with patients carrying the major allele [49] , and mice lacking CNS expression of Erbb2 and Erbb4 exhibit reduced dendritic spine density in frontal cortex pyramidal neurons [50] . Furthermore, kalirin-7 has been shown to be essential for 5-HT2A receptor-induced dendritic spine growth [44] . Antagonism of the 5-HT2A receptor is considered to be an important mechanism of the action of atypical antipsychotic drugs [51] , and schizophrenic patients consistently exhibit decreased levels of these receptors in several cortical regions [52] . We have previously demonstrated that Kalrn null mice have decreased spine number and dendritic arborization as compared with wild-types [18] , [21] , and we show here that they have thinner temporal association cortices. Interestingly, the human subjects carrying this variant have a thinner cortex in the STS. The STS is part of a network that includes the medial prefrontal cortex and amygdala and is involved in aspects of social cognition, including empathy and theory of mind. Patients show abnormal activation of this network during tasks involving the rating of emotional valence in facial expression [53] , and flat affect item score is negatively correlated with performance on these tasks [54] . While the scope of our analyses is limited by statistical power and does not demonstrate a causal relationship between p.D1338N and specific endophenotypes in carriers, our published and current data on Kalrn knockout mice may fill in the gap to some extent. Mouse knockout data suggest a causal relationship between reduced kalirin function and the regulation of both neuropil size and cortical morphology [18] , [21] . As such morphological alterations are reminiscent of the structural abnormalities seen in schizophrenic patients [55] , [56] , the role of kalirin in regulating cortical thickness in humans and animal models should be explored further. During normal development, cortical pyramidal neurons undergo a period of synaptic pruning during adolescence to refine connections before reaching a steady state level in adulthood [57] . This pruning is exaggerated in schizophrenia, and diminished synaptic density, along with less extensive dendritic arborization and smaller pyramidal neuron soma size, is thought to be one of the cellular morphological changes responsible for the decreased cortical grey matter observed in patients [58] , [59] , [60] . Postmortem analyses of brains from schizophrenia patients also demonstrate a reduction in the density of pyramidal neuron dendritic spines in several regions of the cortex, including the dorsolateral prefrontal cortex, the anterior cingulate cortex and the superior temporal gyrus [23] , [61] . There are important caveats in this study. It should be noted that neither causality nor an association between the p.D1338N variant and any particular phenotype are established in this particular case, due to only two identified carriers. A more definitive test of association would require a large population case–control sample. Nevertheless, our study is one of the first to demonstrate that rare putatively deleterious variants in KALRN can lead to phenotypic changes relevant to schizophrenia. Our results are significant in the context of known supporting evidence for the association of both common and rare variants in KALRN with schizophrenia. The most significant association of a common variant in KALRN in the Psychiatric Genomics Consortium schizophrenia GWAS data set had a P -value of 5 × 10 −4 (ref. 62 ). Although the associations of common KALRN variants with schizophrenia have not reached genome-wide significance, they have been observed in other previous GWAS using different ethnic samples [63] , [64] . Resequencing KALRN in a Japanese sample further suggested that rare (MAF<1%) putatively functional missense SNPs may also contribute to schizophrenia risk [22] . Finally, the preliminary, uncorrected STS finding should be treated with caution. The effect of KALRN on cortical thickness may be relatively weak therefore requiring more subjects for increased statistical power. It should be noted that there have been no single rare coding SNPs that are identified to show a statistically significant association with schizophrenia, even in large exome-sequencing projects [25] , [26] . This does not exclude the possibility that some rare functional variants in certain genes do contribute to susceptibility, and intriguingly, rare coding variants are found to be enriched in synaptic genes [25] , [26] . Our study focuses on the functionality of the KALRN gene and one of its variants, rather than association evidence. We have shown that relationships could, in principle, be drawn between rare genetic sequence variants and neuroimaging and diagnostic phenotypes, given the appropriate number of subjects. Knowledge about the cellular and circuit-level impact of rare genetic variants in human subjects may in future point to disease mechanisms: specific molecular domains or functions, such as enzymatic domains, protein–protein interaction motifs or phosphorylation sites, affected by amino acid changes could provide clues to the downstream/upstream members of the pathway. When done at a suitable scale, this approach may provide insight into the pathogenesis of mental disorders. The approach we have taken could be a blueprint for larger scale studies that combine human genetics, cellular and molecular analysis of impact of mutations, and analysis of cognitive, behavioural and neuromorphometric measures in carriers. Human subjects Study participants were recruited through the Conte Center for the Neuroscience of Mental Disorders at Washington University in St. Louis. Participants included individuals with schizophrenia based on Diagnostic and Statistical Manual of Mental Disorders, Ed IV (DSM-IV-TR) criteria ( n =127), and their non-affected siblings and healthy control participants ( n =246). A subset of these participants also elected to undergo structural MR imaging; their demographic information is as follows: patients (SCZ), n =33, 9 females and 24 males, mean age of 24.3±4.0 years; siblings (SCZ-SIB), n =40, 20 females and 20 males; mean age of 23.6±3.7 years; and controls (CON), n =25, 11 females and 14 males, mean age of 20.3±4.9 years. Details of the recruiting process are discussed elsewhere [65] , [66] . All patients provided signed consent, and all activities and procedures were approved by the Washington University in St. Louis Institutional Review Board. Genomic DNA sequencing PCR amplification of KALRN exons 23–28 and adjacent intronic regions from genomic DNA samples from 127 individuals with schizophrenia and 246 siblings and controls, followed by resequencing and automated indel/SNP analysis, was performed by Beckman Coulter Genomics (Danvers, Massachusetts) on an ABI3730 capillary sequencer. PCR primer sequences are listed in Supplementary Table 3 . Primary neuronal cultures High density cortical neuron cultures were prepared from Sprague–Dawley rat E18 embryos as described previously [67] . Pooled cortices were minced and cells were dissociated in a papain solution containing DNAseI, L -cysteine and EDTA (all from Sigma-Aldrich, St. Louis, Missouri). Cells were further dissociated mechanically and then strained, followed by counting of viable cells. Neurons were plated at a density of 3 × 10 5 cells per well onto coverslips coated with poly-D-lysine (0.2 mg ml −1 , Sigma-Aldrich) in 12-well plates, in plating media (feeding media plus 5% fetal calf serum). After 1 h, the media were changed to feeding media (neurobasal media supplemented with B27 (Life Technologies, Grand Island, New York) and 0.5 mM glutamine). Then 200 μM D,L-2-amino-5-phosphonovalerate (Abcam, Cambridge, Massachusetts) was added to the media 4 days later. Plasmid transfections The plasmid encoding myc-kalirin-7, generated by subcloning of rat kalirin-7 cDNA pSCEP.Myc and then into pEAK10.His, was described previously [14] . The D1338N kalirin-7 variant was created by site-directed mutagenesis using the QuickChange II XL mutagenesis kit (Agilent Technologies, Santa Clara, California). The sequence of the forward mutagenesis primer was 5′-GGCAACATCCAAGAGATCTACAATTTCCATAACAACATC-3′. Cortical neurons (DIV 24–26) were transfected with 4–6 μg of the appropriate cDNAs for 4 h in neurobasal medium in the presence of Lipofectamine 2000 according to the manufacturer’s protocol. COS-7 and hEK-293 cells were grown to ~40% confluency in Dulbecco’s modified Eagle’s medium with 10% fetal bovine serum and penicillin/streptomycin. Cells were then transfected with appropriate cDNAs in Dulbecco’s modified Eagle’s medium without antibiotics or serum using Lipofectamine 2000. Cells were transfected when they reached ~40% confluency and were ~95% confluent at the time of collecting. Rac1 activation assay Transfected hEK-293 cells were collected when they reached ~95% confluency. Active Rac1 levels were assessed using a Rac1 Activation Assay Kit (Millipore, Billerica, Massachusetts) following the manufacturers’ protocol with normalization to total Rac1 as described previously [17] . Antibodies against c-myc (1:500, Santa Cruz Biotechnology, Dallas, Texas) and β-actin (1:4,000, Sigma-Aldrich) were used to control for levels of exogenously expressed protein. Blots were then analysed with ImageJ [68] . Membrane ruffling analysis Analysis of membrane ruffling, a process induced by actin polymerization, was performed in COS-7 cells expressing either wild-type or mutant myc-tagged kalirin-7. Following fixation, cells were immunostained with an anti-myc antibody (Santa Cruz Biotechnology), and F-actin was visualized by incubation with Oregon Green 488-conjugated phalloidin (Life Technologies). Cells expressing myc-tagged protein were imaged using a confocal microscope (Zeiss LSM5 Pascal), and images were analysed using ImageJ. A membrane ruffle was defined as an actin-rich undulating membrane protrusion folding back from the adherent surface of a cell. Analysis of sequence variants in neurons Quantitative analysis of spine number and morphology (area, breadth and length) in cortical pyramidal neurons overexpressing the wild-type KALRN or its associated mutants was performed using an approach we have described previously [16] , [17] , [21] , [44] . Cortical neurons cultured on coverslips of postnatal age DIV 24–26 (corresponding to adolescence) were transfected with pEGFP-N2 (Clontech, Mountain View, California) to express green fluorescent protein (GFP) to visualize cell morphology, either alone or together with myc-tagged kalirin-7 for 48 h. Neurons were then fixed and immunostained to visualize spine morphology. Briefly, neurons were fixed with 4% formaldehyde in 4% sucrose/phosphate buffered saline (PBS), followed by ice-cold methanol. After permeabilization and blocking in a solution of 2% normal goat serum/0.1% Triton X-100/PBS, neurons were incubated with an antibody against GFP (1:1,000, Millipore), and an anti-myc antibody (1:1,000, Santa Cruz) to visualize myc-tagged kalirin-7. Neurons were then washed, incubated with Alexa-Fluor 488- and Alexa-Fluor 568-conjugated secondary antibodies, and mounted onto slides with ProLong Gold Antifade mounting medium. Neurons transfected with the mutation construct were compared with neurons expressing the wild-type gene or GFP only. Expression levels of exogenous protein were normalized to GFP, and only cells that express equal levels of exogenous protein, with consistent subcellular targeting, were analysed. Healthy neurons expressing both GFP and myc-tagged protein were imaged using a 63 × oil immersion objective on a confocal microscope (Zeiss LSM5 Pascal). Z stacks of three to eight images, averaged four times, were taken at 0.37-μm intervals, with a 1,024 × 1,024 pixel resolution at a scan speed of 3 s per section. Cultures that were directly compared were stained and imaged simultaneously. Following reconstruction of two-dimensional maximum projection images, spines were manually outlined, and length, width, area, density were measured in MetaMorph software (Molecular Devices, Sunnyvale, California) and subjected to statistical analysis (Student's t -test). For each condition, a 100-μm dendritic region from each of the 10–20 neurons each from three experiments were analysed. Nissl staining of mouse brains Mice carrying the Kalrn null mutation were generated by replacing exons 27 and 28 of the Kalrn gene with a neo cassette, and have been described previously [18] , [21] . Twelve-week-old mice were anaesthetized with a ketamine/xylazine mixture and perfused transcardially with PBS followed by 4% paraformaldehyde in PBS. Brains were removed, postfixed overnight in 4% paraformaldehyde/PBS, and cryoprotected in 30% sucrose/PBS. Brains were then cryosectioned at 50 μm and mounted on slides. Slides were passed through a graded series of ethanol solutions before being stained with a solution containing 0.625% cresyl violet acetate and 0.375% acetic acid. Slides were then dehydrated and mounted with Permount (Fisher Scientific, Pittsburgh, Pennsylvania). Cortical neuropil analysis Cortical neuropil in mice was quantified using semiautomatic image analysis. The temporal association area from five to six Nissl-stained sections 300 μm apart between bregma −1.82 mm and −3.40 mm, on either side of the midline, were imaged with a × 10 objective (NA 0.17, lateral resolution 0.633 μm per pixel). Analysis was performed remotely using ImageJ, with the experimenter blind to conditions. Images of layer 2/3, 4 and 5 were first thresholded to separate neurons from background. Because of possible variations in staining, images were thresholded automatically on a per-image basis. Images were then made into binary images, and glia were excluded by filtering objects smaller than 100 μm. The density of neuronal cell bodies in each image was quantified for each genotype, and neuropil size was defined as the percent of the area of each image not occupied by cell bodies. Both hemispheres from five to six sections were analysed from three to four mice per genotype. MR image collection and processing T 1 -weighted MPRAGE scans were collected on a Siemens 3T TIM TRIO imaging system (Siemens Medical Systems, Malvern, Pennsylvania) with 1 mm × 1 mm × 1 mm resolution. The MRI scans were processed with the Freesurfer (FS) image analysis suite release 4.1.0 (ref. 69) [69] ( http://surfer.nmr.mgh.harvard.edu ), which produced surface tessellations at the grey/white matter interface and the grey/CSF interface. FS provided 72 cortical regions of interest based on a standard parcellation atlas [70] , along with measures of cortical grey matter thickness (mm) for each of these regions using embedded FS algorithms. Statistical analysis Differences between the KALRN -variant-bearing individual with schizophrenia (KALRN-SCZ) and SCZ population were evaluated by generating standard ( Z ) scores for each cortical parcellation on the cortical thickness. Significance was defined as P <0.05. Due to the exploratory nature of this analysis, scores were not corrected for multiple comparisons. Sign tests were performed to determine the relative placement of the KALRN-SCZ raw score ( x K ) in relation to the SCZ and CON mean values. Sign was evaluated by applying the following: where x K is the KALRN-SCZ raw score, and μ SCZ and μ CON are the schizophrenic and control population means, respectively. If , then sign=1, denoting the KALRN-SCZ value for that anatomical region and measure, x K , is further away from μ CON than μ SCZ is from μ CON in either the positive or negative direction. If , then sign=−1, which signified a value of x K that is closer to μ CON than μ SCZ is to μ CON . As we were interested in values of x K that were accentuations of the SCZ phenotype, that is, deviations from μ CON in the extreme, we identified areas and measures of interest as those where P ( x K )<0.05 and sign=1. This process was repeated to establish similar relationships between the KALRN -variant-bearing sibling (KALRN-SIB) and the SCZ-SIB population. How to cite this article: Russell, T. A. et al. A sequence variant in human KALRN impairs protein function and coincides with reduced cortical thickness. Nat. Commun. 5:4858 doi: 10.1038/ncomms5858 (2014).